Seismic reflection data support episodic and simultaneous growth of the Tibetan Plateau since 25 Myr The spectacular topography of the Tibetan Plateau is the result of collision between India and Eurasia over some 50 Myr, but how the plateau grew to its present size remains a topic of debate. Work along its eastern margin suggests a two-stage uplift (thus growth of the plateau) since 30–25 Myr. Here we report high-resolution seismic reflection and drill core results from the southern Tarim Basin that indicate a similar pattern for the northern margin of the plateau. The data suggest that uplift in northern Tibet started at ~23 Myr from near sea level, with the first episode finished by ~10 Myr, followed by a post-5-Myr episode of rapid uplift along the present plateau margin. The growth of the Tibetan Plateau after the Eocene thus appears to have been episodic in nature, and near-synchronous along both eastern and northern margins. Opinions regarding the rise of the Tibetan Plateau range from synchronous plateau-wide uplift [1] to stepwise northward plateau growth [2] . Recent work along the eastern margin of the plateau demonstrates two episodes of rapid uplift: one from 30 to 25 Myr and another from 15 to 10 Myr (ref. 3 ), which appears to favour the episodic plateau growth model. Work along the West Kunlun Range at the northwest margin of the Tibetan Plateau, however, has led to diverse conclusions, ranging from three-episode uplift [4] to a single post-4.5 Myr uplift [5] . Estimations for the initiation of uplift range from ~46 Myr to ~3 Myr (refs 4 , 5 , 6 , 7 , 8 , 9 , 10 , 11 , 12 , 13 ) based on a variety of approaches: ~46 Myr based on stratigraphic and sedimentary analysis [6] ; ~37−30 Myr based on chronology and lithostratigraphy [2] , [7] , [8] ; ~25–15 Myr based on fission track dating [9] , thermochronological results [10] and Nd isotopic analysis of dust [11] and ~4.5 Myr or younger based on magnetostratigraphic and palaeo-environmental analyses [4] , [5] , [12] , [13] . No previous attempt has been made to constrain the uplift history using the subsurface stratigraphic record in the desert-covered Tarim Basin apart from a mentioning in a regional overview [14] . The continental lithosphere of the Tarim Block underthrusts northern Tibet to its south [15] , [16] , [17] , [18] , with up to 12 km thick of Cenozoic foreland basin deposits accumulated along southern Tarim due to the loading of the plateau [6] . These deposits provide a unique record of the history of the mountain building [19] . Here we report the results of two high-quality petroleum prospecting seismic lines and two drill holes from the foreland basin in southwestern Tarim, which enable us to independently estimate the timing and rate of plateau uplift along the northwestern margin of the Tibetan Plateau. Our work points to two episodes of uplift from near sea level since ~23 Myr, and we conclude that the growth of the Tibetan Plateau since the Eocene has been episodic and near-synchronous along its eastern and northern margins. Geological setting Our study region is located at the piedmont of the West Kunlun Range, which marks the northwestern edge of the Tibetan Plateau ( Fig. 1 ). The West Kunlun orogenic belt is bounded to the south by the Karakax Fault and to the north by the Tekilik Fault [17] , [20] . It is characterized by high topographic relief with elevation of up to 6,500 m, 4,000–5,000 m higher than the average elevation of the southwestern Tarim foreland basin. The Tarim Block to the north has an Archaean to Proterozoic crystalline basement. Shallow-marine limestone and calcareous shale were deposited for much of the time from the Cambrian until at least ~25 Myr, and could be as late as ~15 Myr [10] , [21] . Sequence stratigraphic boundaries and their ages within the study region are based on the fossil record and lateral correlations with type sections of the Tarim basin [22] , [23] . Palaeocene and Eocene strata developed in restricted areas only in the Tarim Basin [22] , and drill-hole data reveal a depositional hiatus between the Permian and the Oligocene in the study region. The Cenozoic strata here exhibit a general coarsening upward trend ( Fig. 2 ). The ~130-m-thick Oligocene Bashiblake Formation (E 3 1 ) marine carbonate platform deposits [13] , [23] mark the end of marine carbonate deposition in the basin. The Miocene Wuqia Group (N 1 ) consists of clastic tidal flat (the Keziluoyi N 1 1 and Anjuan N 1 2 formations) and mixed flat facies (the Pakbulak Formation N 1 3 ), with lithology including a series of marine and terrestrial sandstone, shale and mudstone. This group exhibits a progressively higher-energy depositional environment [22] , [23] . The Pliocene Artux formation (N 2 ) comprises dominantly fluvial and alluvial-fan deposits, marking the emergence of the continent above sea level. This was followed by the deposition of the Pleistocene Xiyu formation (Q) alluvial-fan conglomerates intercalated with lenses of siltstone [22] , [23] , [24] ( Fig. 2 ), indicating that the uplifted West Kunlun orogen was by then adjacent to the study region. 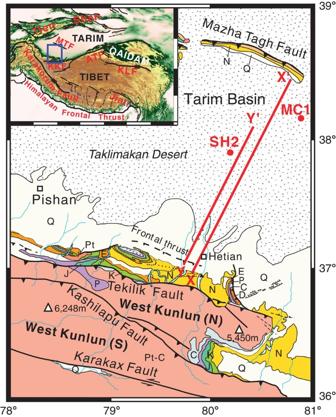Figure 1: Regional map. Simplified geological map of the West Kunlun Range and adjacent areas (after22), showing the location of the two seismic reflection transects (red lines). Red dots show the locations of the two drill holes: SH2 (Shenghe2) and MC1 (Macan1). Inset shows the tectonic framework with relative topography after (ref.29), where the blue rectangle marks the location of the study region. Ages of geological units: Pt—Proterozoic; D—Devonian; C—Carboniferous; P—Permian; E—Paleogene; N—Neogene; Q—Quaternary (mainly Pleistocene). ATF=Altyn Tagh Fault; KKT=Karakax Fault; KLF=Kunlun Fault; MTF=Mazha Tagh Fault. Figure 1: Regional map. Simplified geological map of the West Kunlun Range and adjacent areas (after 22 ), showing the location of the two seismic reflection transects (red lines). Red dots show the locations of the two drill holes: SH2 (Shenghe2) and MC1 (Macan1). Inset shows the tectonic framework with relative topography after (ref. 29 ), where the blue rectangle marks the location of the study region. Ages of geological units: Pt—Proterozoic; D—Devonian; C—Carboniferous; P—Permian; E—Paleogene; N—Neogene; Q—Quaternary (mainly Pleistocene). ATF=Altyn Tagh Fault; KKT=Karakax Fault; KLF=Kunlun Fault; MTF=Mazha Tagh Fault. 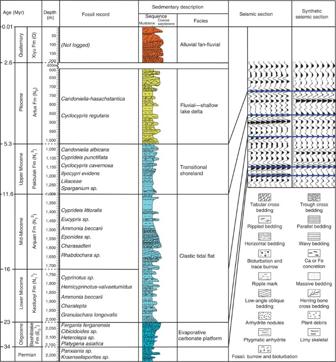Figure 2: Stratigraphic column. Data are from well MC1 located to the north east of the study area, compiled from (ref.23). Quaternary strata cut by the top ~500 m of the drill hole were not logged. Logging of synthetic seismic records of well MC1 is comparable to seismic reflection data, and both consistently show layer interfaces of E31/N11, N11/N12, N12/N13and N13/N2strata. Sedimentary facies and palaeontological information are from regional compilations by (refs22,23,25). Full size image Figure 2: Stratigraphic column. Data are from well MC1 located to the north east of the study area, compiled from (ref. 23 ). Quaternary strata cut by the top ~500 m of the drill hole were not logged. Logging of synthetic seismic records of well MC1 is comparable to seismic reflection data, and both consistently show layer interfaces of E 3 1 /N 1 1 , N 1 1 /N 1 2 , N 1 2 /N 1 3 and N 1 3 /N 2 strata. Sedimentary facies and palaeontological information are from regional compilations by (refs 22 , 23 , 25 ). Full size image Seismic reflection data and foreland basin geometry Seismic reflection and drill-hole data were acquired in the foothills of the West Kunlun Range and the southwestern Tarim foreland basin for petroleum prospecting by the Shengli Oilfield Company during 1997–2000, and the data of two transects (X-X′ and Y-Y′) and two wells (MC1 and SH2; for locations see Fig. 1 ) were provided to the Ocean University of China for scientific purposes under a scientific cooperation agreement. As the two parallel transects, ~10 km apart, show similar structures ( Fig. 3 ), and transect BB′ has a higher resolution, we combined them into a single transect to strengthen the image with transect Y-Y′ joined with the northeastern section of transect X-X′ using the ProMax Oil software. The joint seismic transect was converted to a depth-migrated section constrained by synthetic seismogram of VSP velocity of wells MC1 and SH2 ( Fig. 4a ). 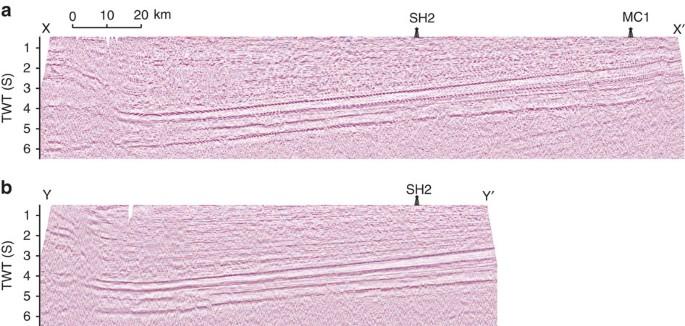Figure 3: Original seismic data. (a) Seismic reflection results along transect X-X′. The projected locations of wells MC1 and SH2 on the transect are shown. (b) Seismic reflection results along transect Y-Y′, with the projected location of well SH2 shown. Figure 3: Original seismic data. ( a ) Seismic reflection results along transect X-X′. The projected locations of wells MC1 and SH2 on the transect are shown. ( b ) Seismic reflection results along transect Y-Y′, with the projected location of well SH2 shown. 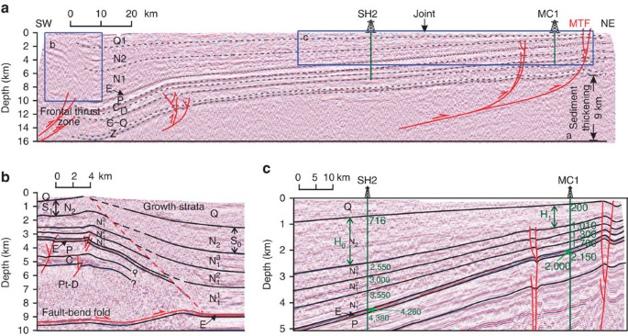Figure 4: Interpreted seismic data and basin geometry. (a) Geological interpretation of the composite seismic reflection transect across the front of the West Kunlun thrust belt and its foreland basin, using results from two seismic profiles X-X′ and Y-Y′ (Fig. 3; seeFig. 1for locations) with the junction marked by ‘Join’. Wells MC1 and SH2 are projected onto the plane of the transect. Dotted lines are interpreted stratigraphic boundaries. The surface of the basement shows a 9-km subsidence towards the thrust belt. (b) Detailed interpretation of seismic reflection data across the frontal thrust, showing a fault-bend fold and growth strata. (c) Detailed foreland basin stragraphic interpretation as constrained by drill holes SH2 and MC1. Numbers in green are depths in metres. Both (a) and (c) show that the growth strata are post-Oligocene (marked as E) in age. Pt—Proterozoic; Z—Neoproterozoic;ε– Cambrian; O—Ordovician; D—Devonian; C—Carboniferous; P—Permian; E—Paleogene; N—Neogene; Q—Quaternary. Full size image Figure 4: Interpreted seismic data and basin geometry. ( a ) Geological interpretation of the composite seismic reflection transect across the front of the West Kunlun thrust belt and its foreland basin, using results from two seismic profiles X-X′ and Y-Y′ ( Fig. 3 ; see Fig. 1 for locations) with the junction marked by ‘Join’. Wells MC1 and SH2 are projected onto the plane of the transect. Dotted lines are interpreted stratigraphic boundaries. The surface of the basement shows a 9-km subsidence towards the thrust belt. ( b ) Detailed interpretation of seismic reflection data across the frontal thrust, showing a fault-bend fold and growth strata. ( c ) Detailed foreland basin stragraphic interpretation as constrained by drill holes SH2 and MC1. Numbers in green are depths in metres. Both ( a ) and ( c ) show that the growth strata are post-Oligocene (marked as E) in age. Pt—Proterozoic; Z—Neoproterozoic;ε– Cambrian; O—Ordovician; D—Devonian; C—Carboniferous; P—Permian; E—Paleogene; N—Neogene; Q—Quaternary. Full size image The foreland deposits dip gently to the southwest, and thicken by ~9 km over the distance of ~170 km, indicating a clear image of the wedge-shaped foreland basin geometry ( Fig. 4a ). The folds and thrusts revealed in the transect show that the thrust belt has been progressively incorporating the foreland basin over time. Syntectonic growth strata began to accumulate in the early Miocene, with the Keziluoyi Formation, a tidal-flat succession, marking a sharp break from the underlying marine platform carbonates of the Bashiblake Formation (E 3 1 ) [23] . Marine foraminifera Ammonia beccarii and ostracod Hemicyprinotus valvaetumidus of the Keziluoyi Formation are found in both well MC1 and outcrops in the southwestern Tarim Basin [22] , [25] . An age range of ~23–16 Myr is assigned to the formation following the recent geological timescale [26] . Likewise, fossil-constrained ages bracket the Anjuan Formation at 16–11.6 Myr, the Pakabulake Formation at 11.6–5.3 Myr and the Artux Formation at 5.3–2.6 Myr (refs 22 , 23 ) ( Fig. 2 ). Time for the onset of uplifting in the West Kunlun Range The change in sedimentary environment from a marine carbonate platform in the Oligocene (the Bashiblake Formation, E 3 1 ) to a clastic tidal flat in the early Miocene (the Keziluoyi Formation, N 1 1 in Figs 2 and 4b,c ) marks the beginning of foreland basin development due to the formation of the proto-West Kunlun Range at the northern edge of the proto-Tibetan Plateau. The estimated ~23 Myr initiation age for the uplift of the proto-West Kunlun Range, based on seismic stratigraphy and the fossil record, is consistent with 22.1–13.7 Myr apatite fission track ages for gneisses in the West Kunlun Range front [9] . It is also consistent with the ~25 Myr age for north-south contraction along the Pamir-West Kunlun Range [27] , the 25–23 Myr ages for large-scale dextral strike-slip movements in northwestern Tibetan Plateau [28] and the 25–20 Myr ages for rapid exhumation at northern Tibet [9] . As the orogen grew higher and possibly also extended to the southern part of the Tarim Basin due to the northward propagation of the Tibetan Plateau, high-energy tidal sediments were deposited (the Anjuan and Pakbulake formations, N 1 2 and N 1 3 ; Fig. 2 ). Since the Pliocene, the sedimentary facies became dominantly fluvial and alluvial fans (the Artux and Xiyu Formations, N 2 and Q; Fig. 2 ). Rates of episodic uplift and basin subsidence A quantitative estimation of differential sedimentation rates in the foreland basin can be made utilizing the high-resolution seismic data ( Figs 4 and 5a , including locations of drill holes), constrained by the drill-hole data and the fossil record ( Fig. 2 ). This allows us to estimate the rates of differential uplift between the two sides of the frontal thrust in the West Kunlun Range ( Fig. 1 ), as well as subsidence rates in the foreland basin. These estimations shed new light on both the episodic nature of plateau propagation and variations in the intensity of orogenic uplift (plateau propogation) with time. 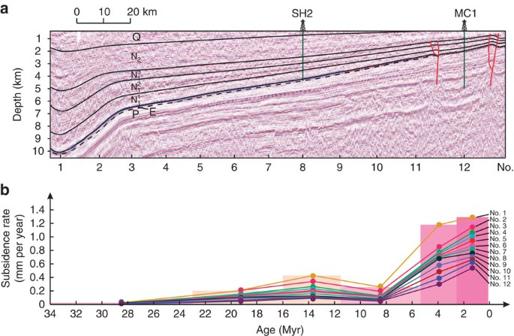Figure 5: Time-space variations in foreland subsidence rate. (a) Stratigraphic interpretation of the composite seismic transect constrained by drill holes MC1 and SH2, showing the geometry of the Cenozoic at foreland basin and older strata. The growth strata of post-Oligocene age, thickening to the southwest, are easily recognizable. Numbers at the bottom of the figure show positions of the 12 locations used for calculating the foreland basin subsidence rates in (b). P—Permian; E—Paleogene; N—Neogene; Q—Quaternary. (b) Calculation results of subsidence rate changes with time for the 12 locations along the seismic transect as shown in (a), using strata thickness as determined by the seismic data calibrated using drill-hole data (Figs 2and3), with age constraints provided by the fossil record (Fig. 2). The shaded columns indicate time intervals for the estimated data points. Calculation results are given inTable 1. Figure 5: Time-space variations in foreland subsidence rate. ( a ) Stratigraphic interpretation of the composite seismic transect constrained by drill holes MC1 and SH2, showing the geometry of the Cenozoic at foreland basin and older strata. The growth strata of post-Oligocene age, thickening to the southwest, are easily recognizable. Numbers at the bottom of the figure show positions of the 12 locations used for calculating the foreland basin subsidence rates in ( b ). P—Permian; E—Paleogene; N—Neogene; Q—Quaternary. ( b ) Calculation results of subsidence rate changes with time for the 12 locations along the seismic transect as shown in ( a ), using strata thickness as determined by the seismic data calibrated using drill-hole data ( Figs 2 and 3 ), with age constraints provided by the fossil record ( Fig. 2 ). The shaded columns indicate time intervals for the estimated data points. Calculation results are given in Table 1 . Full size image We use the thickness variations in the foreland basin to calculate the changing rate of sedimentation with time at different locations in the foreland basin (see locations 1 to 12 marked along the seismic traverse in Fig. 5a ), calibrated by the sedimentation record in wells SH2 and MC1 where the strata thicknesses are marked as H 0 and H 1 , respectively ( Fig. 4c ). Assuming equilibrium subsidence versus deposition rates in the tidal-flat to fluvial/aluvial fan environments, the average deposition (subsidence) rates are given in Table 1 and shown in Fig. 5b . The 12 locations across the foreland basin show a consistent pattern in the change of deposition/subsidence rate with time, with one low peak during the mid-Miocene (~16–11 Myr) and a high peak during the Quaternary (after ~2.6 Myr). The fact that data points inside or close to the orogen (that is, locations 1 and 2) and those away from the orogen (locations 3 to 12) show the same time-variation pattern indicates that the pattern can not be explained by factors such as lithospheric softening within the orogen. The time-variation in deposition/subsidence rate thus most likely reflects changes in the orogenic loading on the lithosphere of the Tarim Block, which would have resulted in isostasy-driven surface uplift at the present northwestern margin of the Tibetan Plateau. The rate estimations for location No. 1 near the depocenter ( Fig. 5 ) are shown in Fig. 6 . It implies that there have been two episodes of rapid uplift along the West Kunlun Range: one in the mid-Miocene (~16–11 Myr) and the other since ~5 Myr, with the latter being significantly more rapid. The peak deposition/subsidence rate for the depocenter was ~0.4 mm per year during mid-Miocene and ~1.3 mm per year for the Quaternary ( Fig. 6 ). Table 1 Results of subsidence rate calculation. 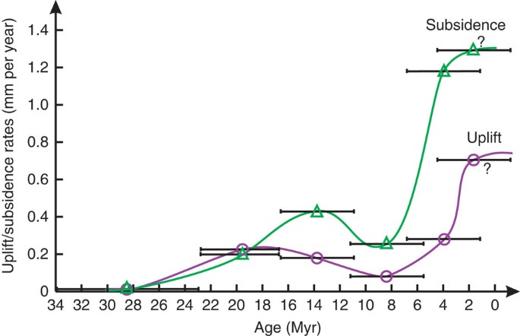Figure 6: Episodic uplift and foreland subsidence. Time variations in the average uplift rate (purple) of the hanging wall of the frontal thrust relative to the footwall, estimated using the thickness contrasts of strata units E31, N11, N12, N13, N2and Q (Table 2), and estimated average subsidence rates (green, using data fromTable 1andFig. 5b), at the depocenter of the foredeep (position 1 inFig. 5a). Full size table Figure 6: Episodic uplift and foreland subsidence. Time variations in the average uplift rate (purple) of the hanging wall of the frontal thrust relative to the footwall, estimated using the thickness contrasts of strata units E 3 1 , N 1 1 , N 1 2 , N 1 3 , N 2 and Q ( Table 2 ), and estimated average subsidence rates (green, using data from Table 1 and Fig. 5b ), at the depocenter of the foredeep (position 1 in Fig. 5a ). Full size image Using the differences in thickness between strata on the two sides of the frontal thrust ( Figs 1 and 4a,b ), we calculated the relative uplift rate on the hanging wall for each time interval by dividing the thickness difference (S 0 −S 1 ) for each unit by the estimated geological duration Δ t . The results also indicate two episodes of rapid uplift along the frontal thrust of the West Kunlun Range: one during the Miocene (~23–12 Myr) with a peak rate of ~0.2 mm per year and the other during the Quaternary (after 2.6 Myr) with a much higher rate of 0.7 mm per year ( Table 2 and Fig. 6 ). Table 2 Results of relative uplift rate at the foothills of the West Kunlun Range across the frontal thrust. Full size table The fact that the relative uplift rate across the frontal thrust shows a comparable periodicity and relative intensity as that suggested by the subsidence/deposition rate estimations ( Fig. 6 ) indicates that (a) the frontal thrust acted broadly synchronously with the main orogenic belt and (b) the interpreted two-episode uplift history, with the post 5 Myr one being much stronger (~3 times that of the earlier one), is a realistic reflection of the uplift history along the West Kunlun Range. The intensity contrast between the two episodes likely indicates that, during the first episode, the front of the proto-West Kunlun orogen at the edge of the plateau was further south from its present position, and it only propagated to its present position during the second episode. Our results therefore suggest that the northwestern edge of the Tibetan Plateau underwent two major episodes of propagation since ~23 Myr: one at ~23–12 Myr and the other since 5 Myr, leading to the region being uplifted from near sea-level [10] to the present height of >6,000 m (~5,000 m relative to the Tarim foreland basin). Such a two-episode uplift history is comparable to the two episodes of rapid cooling events recorded along the eastern margin of the Tibetan Plateau [3] . We therefore conclude that the Tibetan Plateau likely experienced two major episodes of lateral propagation towards both its eastern and northern margins after ~25 Myr: one mostly before 10 Myr and the other mostly after 5 Myr. Such a semi-synchronous plateau expansion model is at variance with both the synchronous plateau-wide uplift [1] and the dominantly northward plateau propagation models [2] . Recent work on both margins also suggest that brittle thickening of the upper crust plays the dominant role in the plateau propagation along those margins [29] , [30] . There is therefore a case for synchronous episodic plateau expansion dominantly through brittle thickening of the upper crust rather than mechanisms like crustal channel flow [31] , [32] . Subsidence rate calculation Subsidence rates at 12 locations along the seismic traverse in the southwestern Tarim foreland basin ( Fig. 5a ) are calculated for the time intervals of the Oligocene (E 3 1 ), the Miocene (N 1 1 , N 1 2 , and N 1 3 ) and the Pliocene (N 2 ) epochs, and the Quaternary (Q) period ( Figs 2 and 4 ). Seismic reflection data show that the syntectonic foreland basin growth strata are above the Oligocene Bashiblake Formation (E 3 1 ) ( Figs 4c and 5a ), consisting of the Miocene Keziluoyi (N 1 1 ), Anjuan (N 1 2 ) and Pakbulak (N 1 3 ) formations, the Pliocene Artux Formation (N 2 ) and the Quaternary Xiyu Formation ( Figs 2 and 5a ). Between wells MC1 and SH2 ( Fig. 4c ) there is an ~60-km separation when projected onto the transect. The thickness of the individual formations increases from north to south: the Bashiblake Formation from 108 to 120 m, the Pakbulak Formation from 300 to 710 m, the Anjuan Formation from 400 to 550 m, the Keziluoyi Formation from 290 to 450 m, the Artux Formation from 810 to 1,834 m and the Xiyu Formation from 1,393 to 1,964 (points 12 and 8 of Fig. 4c ). These correspond to average sedimentation rates of 0.01, 0.04, 0.09, 0.05, 0.30 and 0.54 mm per year for each corresponding time interval at well MC1 (location No. 12), and 0.01, 0.10, 0.13, 0.07, 0.68 and 0.76 mm per year at well SH2 (location No. 8), respectively. These numbers (highlighted in shade) were used for calibrating the rate estimation for the other 10 locations along the transect ( Table 1 and plots in Fig. 5b ). Relative uplift rate calculation The relative uplift rate between the two sides of the frontal thrust at the foothills of the West Kunlun Range is estimated for the time intervals of the Oligocene (E 3 1 ), the Miocene (N 1 1 , N 1 2 , and N 1 3 ), the Pliocene (N 2 ) and the Quaternary (Q) using the difference in strata thickness across the fault (S o and S 1 as in Fig. 4b ) divided by the respective time duration. How to cite this article : Jiang, X.-D. and Li, Z.-X. Seismic reflection data support episodic and simultaneous growth of the Tibetan Plateau since 25 Myr. Nat. Commun. 5:5453 doi: 10.1038/ncomms6453 (2014).